Interaction of bipolaron with the H2O/O2redox couple causes current hysteresis in organic thin-film transistors Hysteresis in the current–voltage characteristics is one of the major obstacles to the implementation of organic thin-film transistors in large-area integrated circuits. The hysteresis has been correlated either extrinsically to various charge-trapping/transfer mechanisms arising from gate dielectrics or surrounding ambience or intrinsically to the polaron–bipolaron reaction in low-mobility conjugated polymer thin-film transistors. However, a comprehensive understanding essential for developing viable solutions to eliminate hysteresis is yet to be established. By embedding carbon nanotubes in the polymer-based conduction channel of various lengths, here we show that the bipolaron formation/recombination combined with the H 2 O/O 2 electrochemical reaction is responsible for the hysteresis in organic thin-film transistors. The bipolaron-induced hysteresis is a thermally activated process with an apparent activation energy of 0.29 eV for the bipolaron dissociation. This finding leads to a hysteresis model that is generally valid for thin-film transistors with both band transport and hopping conduction in semiconducting thin films. Research on organic thin-film transistors (OTFTs) has recently made significant technological progress [1] , [2] , [3] , [4] , [5] , [6] , [7] . However, OTFTs are still inferior to their silicon counterparts in terms of reproducibility and long-term stability. When an OTFT operates with its gate voltage ( V g ) sweeping forwardly (from on to off) and reversely (from off to on), a hysteretic behaviour of its current is frequently observed and the threshold voltage ( V th ) becomes bias-dependent [8] , [9] . Current hysteresis can be a consequence of a variety of causes that can be either of extrinsic character such as interface charge traps [10] , [11] , [12] , bulk traps in gate dielectrics [13] , [14] , [15] , ambient atmosphere [16] , [17] , [18] or of intrinsic origin represented by the bipolaron formation of slow mobile charge carriers especially in conjugated polymers [19] , [20] , [21] . For OTFTs with SiO 2 as gate insulator, silanols on the SiO 2 surface [10] as well as ambient absorbates [16] have been of particular concern. Chakrapani et al. [22] proposed that p -doping of diamond under ambient conditions was due to electron extraction from diamond to the H 2 O/O 2 redox couple. This electrochemistry model was successfully employed by Aguirre et al. [23] to correlate the current hysteresis observed in thin-film transistors (TFTs) with carbon nanotube networks (CNNs) as conduction channel to a reversible electrochemical charge transfer between CNN and the H 2 O/O 2 redox couple, rather than the often discussed mechanism invoking the interaction of the single-walled carbon nanotubes (SWCNTs) with silanol groups present on the SiO 2 surface. Aguirre et al. [23] further suggested that the electrochemical effect should be ubiquitous and not limited to organic semiconductor devices. The mobile charge carriers in low-mobility organic semiconductors are commonly modelled as polarons and their transport is usually limited by interchain hopping. Polarons at high concentrations can form doubly charged bipolarons [19] , [20] , [21] . Bipolarons are immobile owing to an improbable two-carrier hopping at the same time. Thus, formation and subsequent dissociation of bipolarons prompted by V g could cause current hysteresis in OTFTs. However, Coulomb repulsion between two positively charged polarons makes the bipolaron formation unfavourable. Counterions are essential in formation [24] and stabilization of bipolarons [19] . Thus far, the origin of counterions is unclear and has been assumed to be extrinsic dopants [25] or oxygen ions [19] . Therefore, the complex hysteresis phenomenon in OTFTs remains poorly understood despite extensive studies. We embed SWCNTs in poly(9,9-dioctylfluorene-co-bithiophene) (F8T2), a conjugated polymer, to facilitate a systematic investigation of current hysteresis, as they represent two typical semiconducting materials with distinct transport mechanisms: hopping and band transport [26] . Their hysteresis behaviour has been studied, separately, using F8T2-capacitors [24] and CNN-TFTs [27] . We show that by varying the channel length, L , of the composite-TFTs, the transport mechanism spans from SWCNT-dominating band transport along a percolating network to F8T2-dominating hopping on sub-percolating paths. The presence of SWCNTs in F8T2 can effectively reduce L in the sub-percolation regime, although the physical L is much longer [28] . As a result, a significant current enhancement compared with having F8T2 alone in the channel is anticipated. In this report, we demonstrate that the hysteresis in OTFTs is caused by an interaction between bipolaron and the H 2 O/O 2 redox couple. This finding leads to a comprehensive model for hysteresis generally valid for TFTs of both band transport and hopping conduction in semiconducting thin films. Device architecture and channel morphology The schematic structure of a bottom-contact composite-TFT is shown in Fig. 1a . The TFT fabrication is detailed in Methods. The atomic force microscopy image of the composite film in Fig. 1b clearly indicates individual or small bundles of SWCNTs being sparsely embedded in the polymer host. Sharing a similar aromatic structure, the fluorene-based F8T2 strongly interact with and well disperse SWCNTs, thereby leading to a stable F8T2/SWCNT composite [29] , [30] . 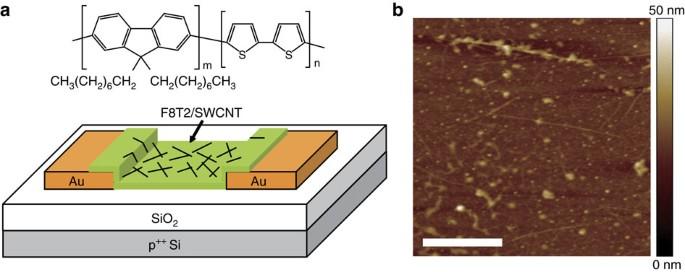Figure 1: Basic device structure. (a) Schematic structure of a back-gate TFT with an F8T2/SWCNT composite film, with the chemical structure of F8T2 shown in the inset. (b) Atomic force microscopy image in height mode of the conduction channel, with a low density of 6 SWCNTs per μm2dispersed in the F8T2 host. The scale bar inbis 1 μm. Figure 1: Basic device structure. ( a ) Schematic structure of a back-gate TFT with an F8T2/SWCNT composite film, with the chemical structure of F8T2 shown in the inset. ( b ) Atomic force microscopy image in height mode of the conduction channel, with a low density of 6 SWCNTs per μm 2 dispersed in the F8T2 host. The scale bar in b is 1 μm. Full size image Electrical characterization The typical transfer characteristics of p -type composite-TFTs for various L are depicted in Fig. 2a . Severe current hysteresis is evident and can be characterized by the difference in V th for forward ( V th f ) and reverse ( V th r ) sweep. The threshold voltages, together with the hysteresis gap (defined as Δ V th = V th r − V th f ), are found to be strongly dependent on L . As illustrated in Fig. 2b , V th f is around −12 V and almost independent of L , while V th r undergoes a continuous negative shift for L >60 μm, resulting in an L -dependent Δ V th . The distinct behaviour of V th f and V th r is discussed later. 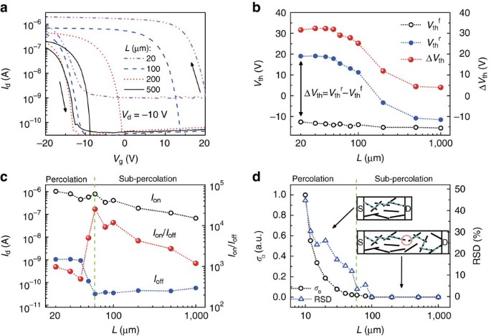Figure 2: Verification of distinct conduction mechanisms. (a) Transfer characteristics of composite-TFTs with variousL, measured atVd=−10 V, with the black arrows indicating theVgsweep directions. The channel width of the TFTs is fixed at 500 μm. (b) Dependence ofVthfandVthras well as of ΔVthonLfor the TFTs ina.VthfandVthrare determined at the sameIdof 10 nA. (c) Variation ofIonandIoffand ofIon/IoffwithLfor the same TFTs. (d) Monte Carlo simulation of sheet conductance (σ□) and the relative s.d. versusLfor a CNN conduction channel. Upper inset shows a percolating SWCNT network in a short channel with the cyan dashed line representing a percolation pathway. In the lower inset, the network no longer percolates in a long channel with the red dotted circle indicating the short break in the CNN that is linked by F8T2 in the composite-TFTs. The black arrows point to the corresponding conduction regimes. The green dashed lines atLC=60 μm incanddindicate the transition from percolation to sub-percolation as the dominant conduction mechanism. Figure 2: Verification of distinct conduction mechanisms. ( a ) Transfer characteristics of composite-TFTs with various L , measured at V d =−10 V, with the black arrows indicating the V g sweep directions. The channel width of the TFTs is fixed at 500 μm. ( b ) Dependence of V th f and V th r as well as of Δ V th on L for the TFTs in a . V th f and V th r are determined at the same I d of 10 nA. ( c ) Variation of I on and I off and of I on / I off with L for the same TFTs. ( d ) Monte Carlo simulation of sheet conductance ( σ □ ) and the relative s.d. versus L for a CNN conduction channel. Upper inset shows a percolating SWCNT network in a short channel with the cyan dashed line representing a percolation pathway. In the lower inset, the network no longer percolates in a long channel with the red dotted circle indicating the short break in the CNN that is linked by F8T2 in the composite-TFTs. The black arrows point to the corresponding conduction regimes. The green dashed lines at L C =60 μm in c and d indicate the transition from percolation to sub-percolation as the dominant conduction mechanism. Full size image As shown in Fig. 2c , the on-current ( I on ) of the composite-TFTs decreases gradually with increasing L , while the off-current ( I off ) experiences a step-like decline by almost two orders of magnitude at a critical channel length L C =60 μm. Thereafter, I off remains fairly constant at ~10 pA. As a result, an I on / I off peak at ~10 4 appears at L C . The abrupt decline of I off (or the resulting sharp increase in I on / I off ) is a signature of the breakdown of the percolating network [28] and the TFT device is now operated in the sub-percolating regime ( Fig. 2d , inset). This experimental observation is verified by Monte Carlo simulation by representing the percolation probability [31] with the normalized sheet conductance ( σ □ ). The simultaneous fall of σ □ and its relative s.d. to zero around L C =60 μm in Fig. 2d suggests that the percolation path breaks altogether at this length. Here, the measured SWCNT density at 6 μm −2 is used as an input parameter in the simulation. With the composite, the non-zero conductance for L >60 μm in Fig. 2c is because of the sub-percolation conduction through the F8T2 host. In the percolation regime, V th r and V th f are independent of L , resulting in a constant hysteresis gap, which is consistent with the results on CNN-TFTs [14] , [17] , [32] . As shown by Aguirre et al. [23] , the following electrochemical reaction is responsible for the hysteresis in CNN-TFTs: Here, the electrochemical potential of the redox couple under the ambient conditions is about −5.3 eV, which lies near the top edge of the valence band of SWCNTs. The electron transfer from SWCNTs to the redox couple is then easy, which is the reason why SWCNTs and most organic semiconductors exposed to air are p -type. In the reverse sweep, the starting positive V g pushes the H 2 O/O 2 electrochemical potential further downward relative to that of SWCNTs. This would promote the electrons being transferred from SWCNTs to the H 2 O/O 2 redox couple to form OH − ions that lead to electrostatic screening of the gate field. In the forward sweep, however, the starting negative V g drives the electrochemical reaction in equation (1) in the reverse direction. This leads to the consumption of OH − ions. Consequently, the change in the amount of absorbed negative charges on the SWCNT surface during the forward and reverse sweeps produces the observed hysteresis. The magnitude of Δ V th depends on the sweep range and rate [17] , [27] , [32] . Use of pulsed measurements with V g pulses of alternating polarities, that is, the AP method, has been reported to distinctively reduce the hysteresis in CNN-TFTs compared with using continuous sweeping [33] , [34] . As shown in Fig. 3a , the hysteresis of a composite-TFT of L =20 μm is almost completely eliminated using the AP method, confirming that the OH − -induced excessive carriers during the positive V g pulse are immediately removed by the subsequent negative pulse. All our devices operating in the percolation regime show hysteresis behaviour consistent with the previous work on CNN-TFTs [34] , [35] , [36] , [37] . In sharp contrast, the AP method causes little difference from the continuous sweeping regarding the hysteresis behaviour of long-channel devices ( L =1,000 μm) ( Fig. 3b ). In these devices, hopping conduction dominates in the sub-percolating F8T2/SWCNT composite. The electrochemical charge transfer occurring between F8T2 and the absorbed H 2 O/O 2 redox couple is therefore predominating over that between SWCNTs and the redox couple. Different from the short-channel composite-TFTs, the channel of the long-channel devices remains in the off-state at V g =0 V for the reverse sweep, resulting in a smaller Δ V th . The H 2 O/O 2 electrochemistry theory alone cannot provide a satisfactory explanation to the hysteresis behaviour in the sub-percolation regime where F8T2 plays a predominating role in channel conduction. Concurrently, the bipolaron mechanism was proposed by Street et al. [19] to explain the bias-stress effect and V th shift in F8T2-TFTs. Immobile bipolarons are suggested to form at negative V g in the reverse sweep during which polarons start to accumulate in the channel. At the beginning of the forward sweep, the bipolaron dissociation is retarded due to a large energy barrier. The retention of the bipolarons at the interface leads to a negative shift of V th . Although the bipolaron mechanism can partly explain the observed hysteresis, it fails to interpret why I off in the reverse sweep is lower than that in the forward sweep since I off should be less affected by the bipolaron formation [19] . Moreover, the formation of bipolarons requires a high concentration of counterions, a critical point seldom discussed in the literature so far. 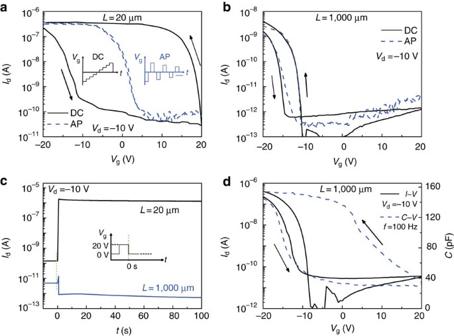Figure 3: Distinct hysteresis behaviour between percolating and sub-percolating devices. (a,b) Transfer characteristics of composite-TFTs withL=20 μm (a) andL=1,000 μm (b) withVgsweeping in DC mode and AP mode. Inset inaschemetically shows the DC and AP mode ofVgsweep. (c) Time dependence ofIdfor the composite-TFTs ofL=20 μm andL=1,000 μm in the first 100 s, in response to a single gate pules ofVg=20 V for 1 s (inset). The green dashed lines indicate the starting point of timing. (d) Forward and reverseVgsweep ofI–VandC–Vcurves of the composite-TFTs ofL=1,000 μm, atVd=−10 V forI–Vand frequency of 100 Hz forC–V, respectively. Figure 3: Distinct hysteresis behaviour between percolating and sub-percolating devices. ( a , b ) Transfer characteristics of composite-TFTs with L =20 μm ( a ) and L =1,000 μm ( b ) with V g sweeping in DC mode and AP mode. Inset in a schemetically shows the DC and AP mode of V g sweep. ( c ) Time dependence of I d for the composite-TFTs of L =20 μm and L =1,000 μm in the first 100 s, in response to a single gate pules of V g =20 V for 1 s (inset). The green dashed lines indicate the starting point of timing. ( d ) Forward and reverse V g sweep of I – V and C – V curves of the composite-TFTs of L =1,000 μm, at V d =−10 V for I – V and frequency of 100 Hz for C – V , respectively. Full size image The BP 2+ –OH − complex model In what follows, a model that invokes the bipolaron formation/recombination in combination with the H 2 O/O 2 electrochemical reaction is proposed to account for the distinct hysteresis behaviour in the sub-percolating composite-TFTs. The polaron–bipolaron equilibrium is represented in equation (2) for the formation of bipolaron–hydroxyl complex, denoted as the BP 2+ –OH − , and in equation (3) for its recombination: Here, R 0 represents a neutral chain segment of F8T2 (ref. 24 ). In the sub-percolating composite-TFTs, electrons are transferred from the composite to the H 2 O/O 2 redox couple at positive V g and {OH − }s are electrochemically generated. The presence of OH − induces polaron accumulation in F8T2 at positive V g . More significantly, two positively charged polarons are, with the assistance of the negative charged OH − , able to overcome the Coulomb repulsion and form the BP 2+ –OH − complex. By transforming most polarons to the immobile BP 2+ –OH − complex, a low drain current, I d , is retained even at negative V g . Recombination of the BP 2+ –OH − complex under sufficiently large negative V g , in accordance to equation (3), leads to release of mobile polarons and increase in I d . This process contradicts Street’s bipolaron theory in that it builds on bipolaron dissociation rather than formation at negative V g in the reverse sweep. In the forward sweep, V th f experiences a slight negative shift, due to the reduction of OH − at negative V g , leading to the observed hysteresis. Furthermore, I off becomes higher than that in the reverse sweep as a result of the retarded bipolaron formation at positive V g in the forward sweep. Therefore, by varying L of the composite-TFTs, the hysteresis mechanism changes from the H 2 O/O 2 electrochemical reaction in the percolation regime to the polaron–bipolaron formation/recombination coupled to the H 2 O/O 2 reaction in the sub-percolation regime. Specifically, V th is governed by the polaron–bipolaron transition and H 2 O/O 2 electrochemical process in the reverse sweep but is less affected in the forward sweep. This explains why V th r strongly varies with L while V th f largely remains constant. The distinct hysteresis behaviour between short-channel and long-channel composite-TFTs can be further demonstrated with a single-pulse measurement. A single positive gate bias pulse for 1 s was applied to two typical devices, one with L =20 μm and the other with L =1,000 μm ( Fig. 3c ). The positive gate pulse is applied to form an ample amount of OH − . They are expected to decay after the pulse. For the shorter-channel device, the H 2 O/O 2 electrochemical process induces holes in the percolating SWCNTs during positive gate pulse, resulting in an abrupt increase in I d by four orders of magnitude followed by a slow decrease with the electrochemistry reaching equilibrium at zero gate voltage. As to the sub-percolating device of L =1,000 μm, the conduction is dominated by hopping in the F8T2 host. The polaron production induced by the H 2 O/O 2 redox couple at the positive gate pulse is quickly transformed to the immobile BP 2+ –OH − complex, resulting in an almost fivefold reduction in I off . These results confirm that the bipolaron formation occurs at positive V g . Although most of the polarons have transformed to immobile BP 2+ –OH − having no contribution to I d , any remaining polarons can respond to capacitance–voltage ( C – V ) measurement and thus resulting in a different hysteresis behaviour. This hypothesis is verified in Fig. 3d , with the C – V and I – V measurements carried out on the same TFT. The C – V measurement was performed at low frequency to avoid the transmission line effect [38] , [39] . The C – V flatband is almost identical to V th f in the forward sweep, as expected. The C – V flatband in the reverse sweep shifts farther than V th r to positive voltage, resulting in a wider capacitance hysteresis gap than Δ V th . The positive flatband voltage shift confirms that the channel is not totally depleted of polarons and the remaining polarons are able to respond the AC small signal superimposed on the DC voltage during the C – V measurement. Dissociation of the BP 2+ –OH − complex under illumination Like excitons in inorganic semiconductors, the BP 2+ –OH − complex is expected to dissociate under illumination according to: Here, h ν is the energy of incident photons. As shown in Supplementary Fig. 1 , V th r significantly shifts to more positive voltage while V th f is less affected during white-light illumination. Thus, a remarkable hysteresis gap comparable with that for the short-channel percolating devices is evident for the long-channel sub-percolating composite-TFTs. Light absorption by SWCNTs does not affect the hysteresis behaviour ( Supplementary Fig. 2 ), while a reference F8T2-TFT shows a similar hysteresis behaviour to the long-channel sub-percolating composite-TFTs ( Supplementary Fig. 3 ). Hence, the illumination helps dissociate almost all immobile BP 2+ –OH − complex formed at positive V g in the reverse sweep into mobile polarons. Further, such illumination-induced hysteresis can be eliminated using the AP method, as for the short-channel devices. The hysteresis behaviour is strongly dependent on the illumination wavelength, λ , as shown in Fig. 4a for the transfer characteristics at different wavelengths. The variation of Δ V th with λ relative to Δ V th in dark is plotted along with the optical absorption spectrum of an F8T2 film in Fig. 4b . The pristine F8T2 film shows a strong absorption in the visible range with two local peaks around 460 and 480 nm, corresponding, respectively, to the π–π* transitions on the F8T2 backbone [40] . The variation of Δ V th with λ correlates well to the absorption spectrum, suggesting that the conduction carriers in the long-channel composite-TFTs in the reverse sweep not only arise from the dissociation of the BP 2+ –OH − complex, but also from the free carriers and excitons created by the bandgap light adsorption. Beyond the absorption edge of the F8T2 film, the small increase in Δ V th is also evident for those at 545 and 578 nm where the F8T2 absorption is negligible. In this beyond-bandgap absorption region, the increase in Δ V th is obviously mainly caused by the dissociation of the BP 2+ –OH − complex. 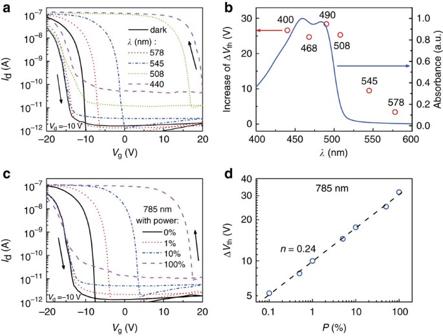Figure 4: Optical response of sub-percolating composite-TFTs ofL=1,000 μm. (a) Typical transfer characteristics measured in darkness and under illumination at different wavelengths. (b) Optical response in terms of increase in ΔVthat several wavelengths of illumination from 400–600 nm (red circles) for the TFT ina. For comparison, the blue solid curve shows the absorption spectrum of an F8T2 polymer thin film. (c) Typical transfer characteristics measured in darkness and under the illumination at 785 nm wavelength with increasing laser power densityP(relative). (d) ΔVth(blue circles) versusPin log–log scale for the TFT inc. The linear fitting in the log–log scale (black dashed line) shows that ΔVthincreases withPfollowing a power function with the indexn=0.24. Figure 4: Optical response of sub-percolating composite-TFTs of L =1,000 μm. ( a ) Typical transfer characteristics measured in darkness and under illumination at different wavelengths. ( b ) Optical response in terms of increase in Δ V th at several wavelengths of illumination from 400–600 nm (red circles) for the TFT in a . For comparison, the blue solid curve shows the absorption spectrum of an F8T2 polymer thin film. ( c ) Typical transfer characteristics measured in darkness and under the illumination at 785 nm wavelength with increasing laser power density P (relative). ( d ) Δ V th (blue circles) versus P in log–log scale for the TFT in c . The linear fitting in the log–log scale (black dashed line) shows that Δ V th increases with P following a power function with the index n =0.24. Full size image In order to further investigate the effects of beyond-bandgap light illumination, a near-infrared laser at 785 nm is used. The transfer characteristics under the 785-nm illumination with relative laser power density, P , are shown in Fig. 4c , yielding a well-correlated relation Δ V th P 1/4 ( Fig. 4d ). This relationship is understood as follows. Variation of Δ V th is equivalent to the shift in V th r . The latter is affected by the variation of polaron density in F8T2, N P , and follows the relation [41] , Δ V th N P . The change in bipolaron density is found to be proportional to the square of the polaron concentration [19] , Δ N BP N P . With reference to equation (4), Δ N BP should be proportional to the number of incident photons or the laser power density, hence, Δ N BP P . These relationships finally yield the experimentally found Δ V th P 1/4 in Fig. 4d and Supplementary Fig. 4 for 633-nm illumination. Finally, the light induced increase in Δ V th beyond the F8T2 bandgap is attributed to the dissociation of the BP 2+ –OH − complex by postulating that the photon energy 1.58 eV for the 785-nm laser is larger than the binding energy of the complex. The hysteresis behaviour is thus a thermally activated process for the long-channel sub-percolating composite-TFTs. Thermal activation energy of the BP 2+ –OH − complex The temperature dependence of Δ V th for the long-channel devices is shown in Fig. 5a . When presented in an Arrhenius plot in Fig. 5b , the mathematical equivalence Δ V th exp(− E a / k B T ) is well followed by all experimental data. Here, E a is the apparent activation energy for the dissociation of the complex, k B the Boltzmann constant, and T the absolute temperature. Further, such thermally-induced hysteresis can be eliminated by characterizing the devices at elevated temperatures, for example, 140 °C, in combination with using the AP method ( Supplementary Fig. 5 ). A good linear fit of the data points in Fig. 5b gives E a =0.29 eV. According to Street et al. [19] , the formation energy of bipolarons would be larger than 0.2 eV for a significant bipolaron concentration at room temperature while it should be above 0.5 eV to completely convert holes to bipolarons. The binding energy of the BP 2+ –OH complex depends on the structure order of the polymer. The regioregular form of conjugated polymers has smaller bipolaron binding energies, which is attributed to the delocalization of the holes arising from the π–π stacking in the two-dimensional structure of the ordered lamellae. The strong π–π interaction between F8T2 and SWCNTs would assist the F8T2 polymer chains to align in parallel with SWCNTs, thereby increasing the polymer conjugation length [42] , [43] . The longer conjugation length, the smaller is the bipolaron binding energy. Hence, use of composite-TFTs is more advantageous in clarifying the origin of hysteresis than using pristine F8T2-TFTs. 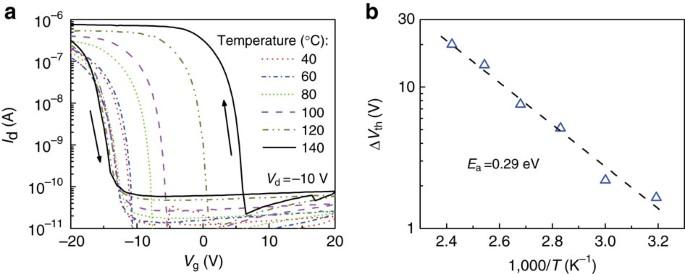Figure 5: Temperature response of sub-percolating composite-TFTs ofL=1,000 μm. (a) Evolution of transfer characteristics with measurement temperature. (b) Arrhenius representation of ΔVthversus reciprocal absolute temperature (blue triangles). The linear fitting in log-linear scale (black dashed line) shows that the process of ΔVthdevelopment is a thermally activated one with an apparent activation energy of 0.29 eV. Figure 5: Temperature response of sub-percolating composite-TFTs of L =1,000 μm. ( a ) Evolution of transfer characteristics with measurement temperature. ( b ) Arrhenius representation of Δ V th versus reciprocal absolute temperature (blue triangles). The linear fitting in log-linear scale (black dashed line) shows that the process of Δ V th development is a thermally activated one with an apparent activation energy of 0.29 eV. Full size image In conclusion, a generic model for current hysteresis in TFTs is proposed. By employing a composite semiconductor comprising SWCNTs embedded in F8T2 films as the conduction channel, we are able to design a unique series of TFTs with channel lengths varying by 2 orders of magnitude in order to confirm the origin of hysteresis in OTFTs. For short-channel devices where the SWCNTs percolate in the conduction channel, the hysteresis behaviour resembles that in CNT-FETs and CNN-TFTs, that is, it is caused by the H 2 O/O 2 electrochemical process interacting with the SWCNTs. Consequently, the hysteresis gap Δ V th is independent of channel length, light illumination and measurement temperature. For long-channel devices in which electronic hoping in the F8T2 matrix prevails for current conduction, the origin of hysteresis is identified to be the formation/dissociation of bipolarons triggered by the H 2 O/O 2 redox reaction. Contrary to the bipolaron mechanism discussed in the literature, the bipolaron is formed at the off-state instead of the on-state and manifests itself in the BP 2+ –OH − complex. The bipolaron-induced hysteresis is sensitive to light illumination even with the beyond-bandgap light. It is also a thermally activated process, with an apparent activation energy of 0.29 eV extracted for the dissociation of the BP 2+ –OH − complex. The established model provides useful guidelines for a deep understanding of hysteresis in TFTs. Solution preparation Both F8T2 (Sigma-Aldrich) and HiPco-SWCNTs (Unidym, average diameter 1.1 nm and average length 1.5 μm) were used as received. F8T2 was first dissolved into toluene (Sigma-Aldrich) in a sonic bath. SWCNTs were ultrasonically added into the F8T2/toluene solution (0.1 mg ml −1 ) followed by centrifugation at 13,300 g for 60 min. The supernatant was then carefully decanted for the TFT fabrication and optical characterization. The ultraviolet-visible absorption spectrum of a thin-film F8T2 drop-cast on a quartz substrate was carried out with a Perkin-Elmer Lambda 750S spectrophotometer. TFT fabrication Heavily doped p -type Si wafers were used as the substrate and back gate, whereas a 100-nm SiO 2 was thermally grown as the gate dielectric. Source and drain electrodes comprising a 50-nm-thick Au layer on top of a 5-nm-thick Ti adhesion layer were defined by means of electron-beam evaporation followed by lift-off. The distance between the source/drain electrodes, that is, the channel length, was varied from 20–1,000 μm. The channel regions were then opened by lithography. For each experiment, one chip was sliced out of the wafer and thin films of F8T2 or F8T2/SWCNT composite were deposited by dip-coating the chip in the polymer solution for 12 h. The chip was then carefully pulled out and baked at 90 °C to remove the residual solvent. The film formed outside the channel was stripped off in acetone along with the photoresist. After blown-dry in N 2 , a 10-min hot-plate baking at 90 °C completed the device fabrication. All the processes were performed under ambient conditions. For the reference CNN-TFT, the chip fabrication was identical to the process described above and the SWCNT conduction channel was formed by dip-coating the chip in the SWCNT/surfactant solution. Device characterization A Keithley 4200 semiconductor characterization system and Agilent 4284A precision LCR metre were utilized for I – V and C – V measurements of the TFTs, respectively. The temperature-varying I – V characterization was performed with a Temptronic temperature controller. All characterizations were usually carried out in dark except for illumination experiments. The illumination experiments were performed at room temperature with a Halogen lamp (12 V, 100 W) filtered through 20-nm-bandpass filters on a Leica microscope (DM2500 M). The optical density of each filtered wavelength was measured with a calibrated Si photodiode (440 nm: 34.2 μW cm −2 , 468 nm: 119 μW cm −2 , 490 nm: 68.3 μW cm −2 , 508 nm: 92.3 μW cm −2 , 545 nm: 141 μW cm −2 , 578 nm: 103 μW cm −2 ). For long-wavelength illuminations, a 17-mW 633-nm He–Ne laser and 250-mW 785-nm near-infrared diode laser were used with various attenuators to reduce the laser intensity. How to cite this article: Qu, M. et al. Interaction of bipolaron with the H 2 O/O 2 redox couple causes current hysteresis in organic thin-film transistors. Nat. Commun. 5:3185 doi: 10.1038/ncomms4185 (2014).